Giant spin-dependent thermoelectric effect in magnetic tunnel junctions Thermoelectric effects in magnetic nanostructures and the so-called spin caloritronics are attracting much interest. Indeed it provides a new way to control and manipulate spin currents, which are key elements of spin-based electronics. Here we report on a giant magnetothermoelectric effect in a magnetic tunnel junction. The thermovoltage in this geometry can reach 1 mV. Moreover a magnetothermovoltage effect could be measured with ratio similar to the tunnel magnetoresistance ratio. The Seebeck coefficient can then be tuned by changing the relative magnetization orientation of the two magnetic layers in the tunnel junction. Therefore, our experiments extend the range of spintronic devices application to thermoelectricity and provide a crucial piece of information for understanding the physics of thermal spin transport. Thermoelectricity has been known since the discovery by T.J. Seebeck in 1821. On one hand, the relation between the thermal and the electrical transport is an essential topic for both fundamental physics and for the future of energy-saving technologies [1] , [2] , [3] , [4] , [5] , [6] . On the other hand, the discovery of the giant magnetoresistance effect and the tunnel magnetoresistance effect (TMR) enhanced the interest of the community for spin-dependent conductivity and gave rise to spintronics and multiple applications [7] , [8] , [9] . Its interplay with thermal conductivity was introduced to describe the conventional Seebeck effect in ferromagnetic metals [10] , [11] , [12] , [13] , [14] , [15] , [16] , [17] , [18] , [19] , [20] , [21] , [22] , [23] , [24] , [25] . The magnetothermoelectric effect has then be studied in magnetic systems such as magnetic multilayers and spin valves [10] , [11] , [12] , [13] , [14] . Moreover, the thermoelectric effect has also been observed in non-magnetic tunnelling devices such as superconductor-insulator-normal metal (or superconductor) tunnel junctions [26] , [27] . Recently, thermal spin tunnelling effect from ferromagnet to silicon has been reported [28] . In regard to magnetic tunnel junction (MTJ), there were theoretical works [29] , [30] , [31] showing magnetothermopower, and Walter et al . [32] reported first the measurements of Seebeck effect in MgO MTJs. Their experiments show that the magnitude and sign of the magneto–Seebeck ratio can be changed by laser power modulation [32] . In this article, we present an experimental discovery of a giant thermoelectric effect in Al 2 O 3 MTJs. The observed mV thermovoltage has promising application for the novel magnetic thermoelectric devices. Experiment set-up The studied MTJ consists of a bottom reference layer Ta(5 nm)/PtMn(25 nm)/Co 90 Fe 10 (2 nm)/Ru(0.8 nm)/Co 90 Fe 10 (3 nm) and a free layer Co 90 Fe 10 (2 nm)/Ni 80 Fe 20 (5 nm)/Ru(4.8 nm)/Au(10 nm) separated by a 2-nm thick amorphous Al 2 O 3 barrier, as shown in Fig. 1a . To generate a temperature difference between the reference layer and the free layer, one electrode lead was heated using the laser beam from a laser diode with a wavelength of 780 nm and a tunable power from 0 to 125 mW. The temperature difference between both sides of the Al 2 O 3 barrier is defined as Δ T , whereas the voltage difference is Δ V . 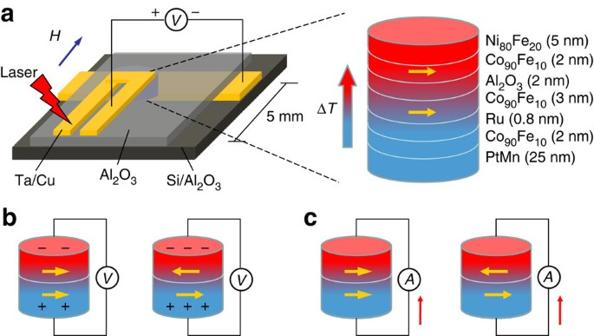Figure 1: Schematic of the experiment. (a) The studied MTJ consists of a bottom reference layer Ta(5 nm)/PtMn(25 nm)/Co90Fe10(2 nm)/Ru(0.8 nm)/Co90Fe10(3 nm) and a free layer Co90Fe10(2 nm)/Ni80Fe20(5 nm)/Ru(4.8 nm)/Au(10 nm) separated by an Al2O3barrier. To generate a temperature difference between both sides of the Al2O3barrier, one electrode lead was heated using the laser beam from a laser diode with the wavelength of 780 nm at a maximum power of 125 mW. The open-circuit voltage was measured by the nanovoltmeter at room temperature (RT) with an applied magnetic field μ0Hup to 0.3 T along the in-plane easy axis. (b) In the presence of the temperature difference ΔTin the MTJ, the generated thermovoltage ΔVdepends on the relative magnetization alignment of the two ferromagnetic layers. (c) The thermotunnel currentIwas measured by the system sourcemeter connecting the MTJ in a closed circuit without applied voltage. In the linear response approximation, the total electric current I in the presence of Δ V and Δ T can be written as [10] , [24] Figure 1: Schematic of the experiment. ( a ) The studied MTJ consists of a bottom reference layer Ta(5 nm)/PtMn(25 nm)/Co 90 Fe 10 (2 nm)/Ru(0.8 nm)/Co 90 Fe 10 (3 nm) and a free layer Co 90 Fe 10 (2 nm)/Ni 80 Fe 20 (5 nm)/Ru(4.8 nm)/Au(10 nm) separated by an Al 2 O 3 barrier. To generate a temperature difference between both sides of the Al 2 O 3 barrier, one electrode lead was heated using the laser beam from a laser diode with the wavelength of 780 nm at a maximum power of 125 mW. The open-circuit voltage was measured by the nanovoltmeter at room temperature (RT) with an applied magnetic field μ 0 H up to 0.3 T along the in-plane easy axis. ( b ) In the presence of the temperature difference Δ T in the MTJ, the generated thermovoltage Δ V depends on the relative magnetization alignment of the two ferromagnetic layers. ( c ) The thermotunnel current I was measured by the system sourcemeter connecting the MTJ in a closed circuit without applied voltage. Full size image where G V is the electrical conductance, and G T is the thermoelectric coefficient related to the charge current response to the heat flux. The thermovoltage Δ V can be measured in an open-circuit geometry, where I =0, as shown in Fig. 1b . Considering equation (1) it leads to Δ V =−( G T / G V )Δ T =− S Δ T , where S = G T / G V is the thermopower (TP) or Seebeck coefficient. Δ V was measured with a nanovoltmeter at room temperature (RT) with a magnetic field H applied along the in-plane easy axis of the free layer. The thermotunnel current was measured by a sourcemeter connecting the MTJ without any applied voltage, that is, a closed circuit, as shown in Fig. 1c . In the closed-circuit geometry, Δ V =0 and thus from equation (1), I = G T Δ T . With those two geometries, the influence of magnetization orientations on both spin-dependent electrical conductivity and thermoelectric effect could be studied. 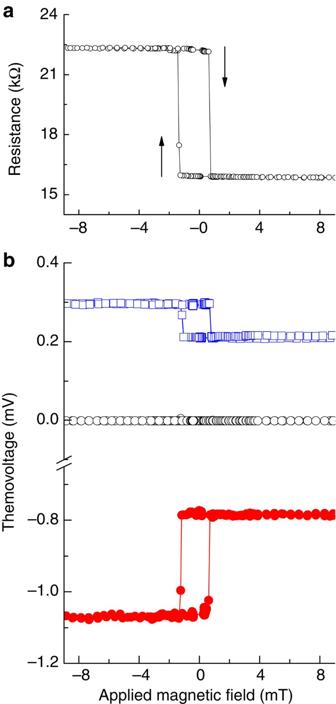Figure 2: Magnetic field dependence of the tunnel resistance and the thermovoltage in a MTJ. (a) Minor loop of the tunnel resistanceRof an Al2O3MTJ with a diameter of 80 μm as a function ofHat room temperature, measured with a 0.1-μA current. The arrows indicate the sweeping direction of the magnetic field. The MTJ has a low resistanceRP=15.9 kΩ for the parallel (P) magnetization alignment, and a high resistanceRAP=22.3 kΩ for the antiparallel (AP) alignment. The TMR ratio is (RAP−RP)/RP=40%. (b) Thermovoltage versus applied field (V–H) minor loops. The voltage across the MTJ is measured in an open-circuit geometry with a laser heating the electrodes. As the laser heats the top lead (solid circle), the temperature of the free layer is higher than that of the reference one, that is, ΔT>0, yielding a negative thermovoltage ΔV, whereas a positive ΔVis observed in the case of the laser heating the bottom lead (open square), that is, ΔT<0. It is noted that the open-circuit voltage is zero in the absence of laser heating (open circle). With sweeping the applied field, ΔVshows a behaviour similar toR.The amplitude of the thermovoltage for the AP alignment, ΔVAP, is larger than that for the P, ΔVP. The ΔVAPcan reach −1.07 mV as heating the top lead with a 125 mW laser power, while the ΔVAPis about 310 μV as heating the bottom lead with the same laser power. The tunnel magnetothermovoltage ratio defined as (VAP−VP)/VPis ~40%, which is similar with the TMR ratio of the MTJ. Magnetothermovoltage measurement in MTJ Figure 2a shows a minor loop of the tunnel resistance R as a function of the in-plane applied field H for an Al 2 O 3 -based MTJ with a diameter of 80 μm. The MTJ has a low resistance R P =15.9 kΩ for the parallel (P) magnetizations alignment, and a high resistance R AP =22.3 kΩ for the antiparallel (AP) magnetizations alignment, showing a TMR ratio ( R AP − R P )/ R P =40%. Figure 2: Magnetic field dependence of the tunnel resistance and the thermovoltage in a MTJ. ( a ) Minor loop of the tunnel resistance R of an Al 2 O 3 MTJ with a diameter of 80 μm as a function of H at room temperature, measured with a 0.1-μA current. The arrows indicate the sweeping direction of the magnetic field. The MTJ has a low resistance R P =15.9 kΩ for the parallel (P) magnetization alignment, and a high resistance R AP =22.3 kΩ for the antiparallel (AP) alignment. The TMR ratio is ( R AP − R P )/ R P =40%. ( b ) Thermovoltage versus applied field ( V – H ) minor loops. The voltage across the MTJ is measured in an open-circuit geometry with a laser heating the electrodes. As the laser heats the top lead (solid circle), the temperature of the free layer is higher than that of the reference one, that is, Δ T >0, yielding a negative thermovoltage Δ V , whereas a positive Δ V is observed in the case of the laser heating the bottom lead (open square), that is, Δ T <0. It is noted that the open-circuit voltage is zero in the absence of laser heating (open circle). With sweeping the applied field, Δ V shows a behaviour similar to R. The amplitude of the thermovoltage for the AP alignment, Δ V AP , is larger than that for the P, Δ V P . The Δ V AP can reach −1.07 mV as heating the top lead with a 125 mW laser power, while the Δ V AP is about 310 μV as heating the bottom lead with the same laser power. The tunnel magnetothermovoltage ratio defined as ( V AP − V P )/ V P is ~40%, which is similar with the TMR ratio of the MTJ. Full size image Then, instead of injecting a current in the MTJ, as sketched in Fig. 1b , the voltage across the MTJ is measured in an open-circuit geometry. The top lead is heated by the laser to generate a temperature difference between the free layer and the reference layer spaced by the Al 2 O 3 barrier. With the top lead heated, the temperature difference is defined as positive Δ T >0. As shown in Fig. 2b , a negative thermovoltage Δ V is detected in this geometry. While sweeping the in-plane applied field, a sudden Δ V increase is observed as the free layer magnetization switches and the magnetization configuration changes from P to AP. In fact, the Δ V versus H hysteresis loop mimics the R versus H loop. Two thermovoltage levels are clearly defined corresponding to the two magnetization alignments (P and AP). The amplitude of the thermovoltage for the AP alignment, Δ V AP , is found to be larger than that for the P, Δ V P . In our case, the Δ V AP can reach up to −1.07 mV while heating the top lead with a 125-mW laser power. The Δ V AP is about 310 μV as heating the bottom lead with the same laser power. This difference can be understood as different material, thickness and size for the top and bottom leads result in different heat conductivity and dissipation. In the case where the laser heats the bottom lead, that is, Δ T <0, then a positive thermovoltage is measured, as shown in Fig. 2b , and an inverse thermovoltage Δ V hysteresis loop is observed. Note that if the laser is turned off or shines the substrate instead of the leads, the thermovoltage decreases to zero and no influence of the applied field is observed. For both top and bottom heating, the tunnel magnetothermovoltage ratio defined as (Δ V AP −Δ V P )/Δ V P is ~40%, which is similar to the TMR ratio. This behaviour suggests that the observed thermoelectric effect mainly results from the thermal spin-dependent tunnelling between both sides of the Al 2 O 3 barrier. Moreover, the thermovoltage of the lead was measured while heating one end with the maximum laser power, and a value <2 μV was obtained. Thus, the thermovoltage of the lead can be neglected considering the measured thermovoltage in the MTJ. 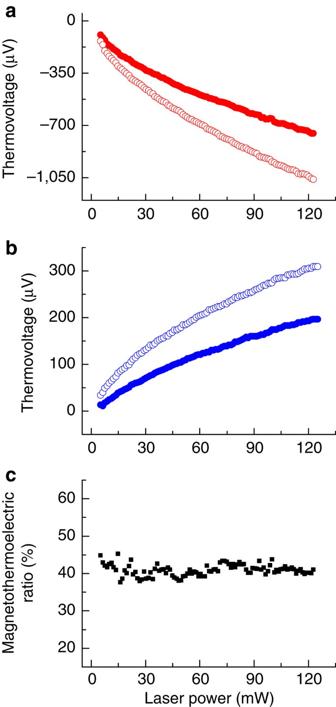Figure 3: Laser power dependences of the magnetic thermovoltage and magnetothermoelectric ratio in the MTJ. The thermovoltage ΔVP(solid circles) and ΔVAP(open circles) as a function of the laser powerPin the cases of heating the top lead (a) and the bottom lead (b). It is found that ΔVPand ΔVAPbehave likeP1/2. (c) The magnetothermovoltage ratio (ΔVAP−ΔVP)/ΔVPas a function of the laser power. It is ~40%, which is very close to the TMR ratio, and is constant with the laser power. Figure 3 shows the thermovoltage Δ V P and Δ V AP as a function of the laser power P in the cases of heating the top ( Fig. 3a ) and the bottom leads ( Fig. 3b ). One can see that the amplitudes of both Δ V P and Δ V AP increase with the laser power. The experimental data, obtained for Δ V P and Δ V AP , are not linear but following a P 1/2 -like behaviour for the top lead and bottom lead heating. In our understanding this P 1/2 behaviour is not the signature of a microscopic process, but rather is due to the dependence of the temperature difference and of the Seebeck coefficient with P . Owing to power dissipation, the temperature difference follows a P α law with α <1, and the Seebeck coefficient is itself a complicated function of the temperature, and thus of P . The magnetothermovoltage ratio (Δ V AP −Δ V P )/Δ V P is 40%, which is close to the TMR ratio, and changes little with the laser power, as shown in Fig. 3c . Figure 3: Laser power dependences of the magnetic thermovoltage and magnetothermoelectric ratio in the MTJ. The thermovoltage Δ V P (solid circles) and Δ V AP (open circles) as a function of the laser power P in the cases of heating the top lead ( a ) and the bottom lead ( b ). It is found that Δ V P and Δ V AP behave like P 1/2 . ( c ) The magnetothermovoltage ratio (Δ V AP −Δ V P )/Δ V P as a function of the laser power. It is ~40%, which is very close to the TMR ratio, and is constant with the laser power. 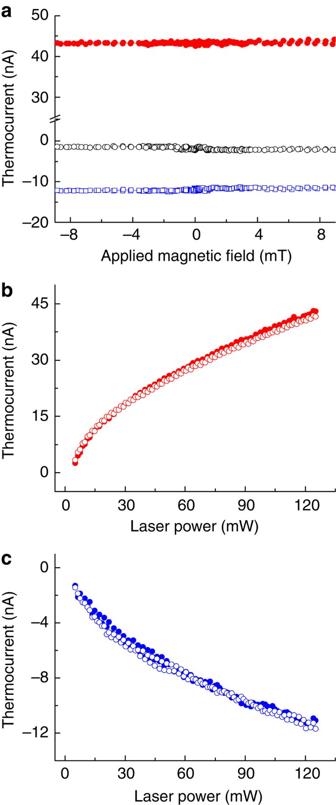Figure 4: Magnetic field and laser power dependence of the thermotunnel current in the MTJ. (a) Thermotunnel current versus applied field (I–H) curves in the cases of heating the top lead (solid circles), the bottom lead (open squares) and without heating (open circles).Iis independent on the magnetization alignments. (b,c) The thermotunnel currentIP(solid circles) andIAP(open circles) as a function of the laser powerPfor heating the top and the bottom leads, respectively. It is found thatIPandIAPare following aP1/2-like behaviour. Full size image Thermotunnel current measurement in MTJ Figure 4a shows the measured thermotunnel current I as a function of H in a closed-circuit geometry, as described above. Without laser heating, the closed-circuit current is around zero. As heating the top lead with a 125-mW laser power, I reaches 43 nA, and I is about −12 nA when the bottom lead is heated by the same laser power. One can see that the thermotunnel current I is independent on the magnetization alignments. However, similarly with the thermovoltage, the laser power dependence of the thermotunnel current also behaves like P 1/2 for both top and bottom leads heating, as shown in Fig. 4b,c . Considering the amplitude, the sign and the magnetic dependence of the measured signal, the possibility of an artefact coming from the known light-induced phenomenon could be ruled out. Figure 4: Magnetic field and laser power dependence of the thermotunnel current in the MTJ. ( a ) Thermotunnel current versus applied field ( I – H ) curves in the cases of heating the top lead (solid circles), the bottom lead (open squares) and without heating (open circles). I is independent on the magnetization alignments. ( b , c ) The thermotunnel current I P (solid circles) and I AP (open circles) as a function of the laser power P for heating the top and the bottom leads, respectively. It is found that I P and I AP are following a P 1/2 -like behaviour. Full size image From the above experimental results obtained in Al 2 O 3 MTJs, one can see that the magnetothermovoltage is proportional to TMR, that is, Δ V P /Δ V AP = R P / R AP , whereas the thermotunnel current is independent on magnetizations relative orientations. As the thermovoltage is given by Δ V =−( G T / G V ) Δ T =− S Δ T , whereas the thermocurrent is given by I = G T Δ T , assuming that for a fixed laser power Δ T is constant for the P and AP configuration, we could define a tunnel TP S , which depends strongly on the magnetization alignment of the two magnetic layers. It leads to the conclusion that the coefficient G T is independent on the magnetization alignments. Consequently, the tunnel magnetothermopower is proportional to TMR in Al 2 O 3 MTJs, that is, S P / S AP =R P / R AP . It should be said that this behaviour is not conventional, as usually the Seebeck coefficient is not dominated only by the resistance. Indeed, the experiments of other groups [32] , [33] show that there is no direct relation between magneto–Seebeck effect and TMR in MgO MTJs, which agree with the ab-initio calculation [31] . To obtain the value of S , the temperature difference between both sides of the tunnel barrier is needed. Unfortunately, it is hard to directly measure a small temperature difference between a 2-nm barrier. The temperature difference between the bottom and top leads was obtained by measuring the temperature of each lead with a k-type thermocouple connected to a nanovoltmeter. As shown in Fig. 5 , for instance with a laser power of 125 mW heating the bottom lead, the temperatures of the leads are about 319 K, whereas the temperature difference between the top and the bottom leads is 300±250 mK. We could conclude that the temperature difference is smaller than 1 K between the top and the bottom leads, which could be much smaller between both sides of the tunnel barrier in the MTJ. It should be noted that only part of the heat goes through the MTJ, and because the size of MTJ is much smaller than that of the leads and the 2-nm thickness of Al 2 O 3 barrier is small comparing with the 60 nm thickness of the whole multilayers, the vertical temperature difference across the 2-nm Al 2 O 3 barrier should be smaller than the one measured between the two leads. For a 125-mW laser power, an upper limit for the temperature difference across the barrier can be estimated to be ~100 mK. Consequently, from the measured 1-mV thermovoltage, we can estimate that the Seebeck coefficients in Al 2 O 3 MTJ should be on the order of 1 mV K −1 or larger, which is large compared with the conventional metals and semiconductors [1] . 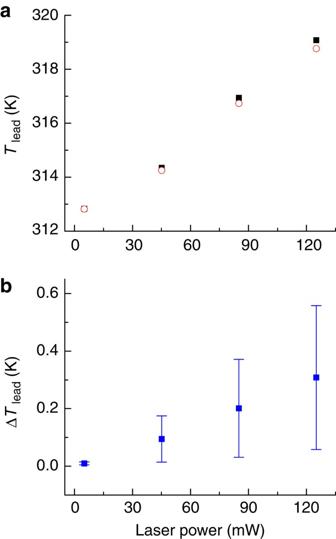Figure 5: Laser power dependence of the temperature difference of the leads in the MTJ. (a) Temperatures of the bottom lead (solid squares) and the top lead (open circles) as the bottom lead was heated for various laser powers. (b) Laser power dependence of the temperature difference between the bottom and the top leads. The error bars of the temperature difference are given by repeating the measurements. Figure 5: Laser power dependence of the temperature difference of the leads in the MTJ. ( a ) Temperatures of the bottom lead (solid squares) and the top lead (open circles) as the bottom lead was heated for various laser powers. ( b ) Laser power dependence of the temperature difference between the bottom and the top leads. The error bars of the temperature difference are given by repeating the measurements. Full size image Walter et al . [32] show the TP in MgO MTJ of 100 (1300) μV K −1 with a 5.3 μV measured thermovoltage and a simulated temperature difference across the barrier of 53 (4.4) mK. Theoretical study by McCann and Fal'co [30] using inelastic magnon model estimates 55 μV K −1 , and the ab-initio theory by Czerner et al . [31] gives values of up to 150 μV K −1 . This means that giant TP can be obtained in an Al 2 O 3 MTJ. In the following, we provide a simple model within the linear response theory that agrees with our experimental results. Note that this explanation does not exclude that this behaviour could result from a very peculiar inelastic scattering of the electrons with phonons or magnons, but in the absence of detailed experimental evidence of this type of process we will use a description based on elastic scattering only and find the particularities needed to explain the experimental data. In such a case, it is possible to express the Onsager coefficient L 11 = G V and L 12 = G T as the moments of order 0 and 1 of the transport function σ ( ), f is the Fermi-Dirac distribution function, and (−e) the electron charge. This approach is well used for bulk thermoelectricity [1] , [27] , [34] and has recently been applied in the context of spin caloritronics in the works by Czerner et al . [31] and Walter et al . [32] The function σ ( ) has the physical meaning of an energy-dependent conductivity for the electrons. The quantities L 11 and L 12 measure, respectively, the value and the slope of the function σ ( ), k B T around the Fermi level. In the case of a P configuration, σ ( ) is given by whereas for an AP configuration, are the spin-up and spin-down density of states (DOS) in the left (L) and right (R) leads. |T σ σ′ | 2 are the tunnelling functions. From S = G T / G V = L 12 / L 11 , it is clear that the TP will be proportional to the resistivity 1/ L 11 , if L 12 is independent of the magnetization orientation, as found in our experiment. In view of equation (2), this requires the slope of the transport function, averaged k B T around the Fermi level, to be the same in the P and AP configuration. Notice that this does not preclude for the values of σ P and σ AP to be different and therefore allow observing a TMR. Unlike for the MgO MTJs, the Jullière model [7] may be appropriate for the Al 2 O 3 MTJs. Therefore, neglecting the energy dependence of the tunnelling functions, the slopes of should then approximately be the same. Our experimental results would be consistent with DOSs written as where are the DOS for an alloy of cobalt with iron, and δρ a spin-independent contribution that can be understood as a resonance. In such a case, with Because spin-up and spin-down DOS of bulk cobalt and iron have small slope at the Fermi level on the scale of k B T , it is a good approximation that it is also true for their alloys, if no special atomic order is created, as in our compounds. The energy dependence and the slopes of σ P and σ AP are then dominated by the one of the resonance δρ , and therefore is independent on the P or AP configuration. Inserting equations (5) and (6) into equation (2), we obtain the Seebeck coefficients To obtain these expressions we have used the low temperature expansion of the Fermi function, and the following definitions . The numerator of equations (7) and (8) describes why the thermocurrent of Fig. 4a is independent of the magnetization alignment, whereas in the denominator we recognize the Jullière expression for the conductance in term of polarizations a L , R . This explains the proportionality observed between the magneto–Seebeck effect and TMR in Fig. 2 . These formula are also consistent with the large value observed for the thermovoltage, if δρ is a very narrow non-magnetic resonance giving rise to a large δρ′ . This could originate, for example, from non-magnetic impurity states, as they are usually narrow. In summary, large thermoelectric effect was observed in the MTJ arising from the temperature difference between both sides of a 2-nm Al 2 O 3 tunnel barrier. The magnetothermovoltage ratio for the P and AP magnetization configuration is similar to the TMR ratio in the Al 2 O 3 MTJ. However, the thermotunnel current is independent on the magnetization alignments. The TP can be estimated to be >1 mV K −1 in the Al 2 O 3 MTJ, which is larger than that in the metal and semiconductor, suggesting that MTJ can be used as a good thermospin device. The thermospin devices can work in an open-circuit without applying any current or voltage. On one hand, the large change in thermovoltage can be obtained in the presence of a temperature difference through controlling the relative magnetization alignment of the two ferromagnetic layers in the MTJ. On the other hand, the magnetothermovoltage can be used to detect the magnetization configuration even in the open-circuit geometry. The exact mechanism may still be discussed, but we are proposing a description based on elastic scattering to explain qualitatively the experimental results. This work extends the understanding of the spin-dependent thermal and electrical transport in nanostructures, and has promising potential for the design and application of thermally driven MTJ. MTJ preparation The MTJ consists of a bottom reference layer Ta(5 nm)/PtMn(25 nm)/Co 90 Fe 10 (2 nm)/Ru(0.8 nm)/Co 90 Fe 10 (3 nm) and a free layer Co 90 Fe 10 (2 nm)/Ni 80 Fe 20 (5 nm)/Ru(4.8 nm)/Au(10 nm) separated by a 2-nm thick Al 2 O 3 barrier. The films were deposited on the 400 nm Al 2 O 3 covered Si wafers in a DC magnetron sputtering system at RT with a base pressure of 2×10 −8 Torr and a deposition pressures of 2–3 mTorr. The Al 2 O 3 barrier was obtained by reactive rf (radio frequency) oxidation of a 2-nm Al layer at a power of 50 W. The films were annealed for 2 h at the temperature of 265 °C and a 1.3-T magnetic field in a N 2 atmosphere oven, and then patterned to circular shape with the diameter varying from 40 to 100 μm using the photolithography and ion mill processes. The 200 nm Cu and 10 nm Ta were used as both the bottom and the top leads. The MTJs were measured using a system sourcemeter. The TMR is around 40±3% and the resistance-area product is about 22±6 MΩμm 2 at RT. Magnetothermovoltage and thermotunnel current measurements To generate a temperature difference between the reference layer and the free layer, the top lead or the bottom lead was heated using a laser beam from a laser diode with a wavelength of 780 nm and a maximum power of 125 mW. The laser spot on the lead is around 5 mm away from the junction. It should be noted that only part of heat pass through the MTJ, because the power is dissipated and the size of the MTJ is much smaller than that of the leads. The thermovoltage was measured by a nanovoltmeter having an internal resistance larger than 10 GΩ in an open-circuit at RT with an applied magnetic field up to 0.3 T along the in-plane easy axis. The thermotunnel current was measured by a sourcemeter having an internal resistance lower than 100 mΩ, connecting the 16 kΩ MTJ in a closed circuit without applied voltage. The thermovoltage of MTJ was also checked by measuring the AC voltage using a lock-in with the same frequency of the AC laser power. The AC measurement shows the similar behaviour with the DC measurement. The temperature difference in between the bottom and top leads was obtained by measuring the temperature of each lead with a k-type thermocouple connected to a nanovoltmeter. To minimize the error, we tried to install the thermocouple as close as possible to the junction. The temperatures of the leads were also checked by measuring the resistance variation of the leads due to laser heating. The Al 2 O 3 MTJs with the diameters varying from 40 to 100 μm were measured and showed similar behaviours. How to cite this article: Lin, W. et al . Giant spin-dependent thermoelectric effect in magnetic tunnel junctions. Nat. Commun. 3:744 doi: 10.1038/ncomms1748 (2012).